MatP regulates the coordinated action of topoisomerase IV and MukBEF in chromosome segregation The Escherichia coli SMC complex, MukBEF, forms clusters of molecules that interact with the decatenase topisomerase IV and which are normally associated with the chromosome replication origin region ( ori ). Here we demonstrate an additional ATP-hydrolysis-dependent association of MukBEF with the replication termination region ( ter ). Consistent with this, MukBEF interacts with MatP, which binds matS sites in ter . MatP displaces wild-type MukBEF complexes from ter , thereby facilitating their association with ori , and limiting the availability of topoisomerase IV (TopoIV) at ter . Displacement of MukBEF is impaired when MukB ATP hydrolysis is compromised and when MatP is absent, leading to a stable association of ter and MukBEF. Impairing the TopoIV-MukBEF interaction delays sister ter segregation in cells lacking MatP. We propose that the interplay between MukBEF and MatP directs chromosome organization in relation to MukBEF clusters and associated topisomerase IV, thereby ensuring timely chromosome unlinking and segregation. Successful segregation of newly replicated DNA requires that all interlinks between the two strands of duplex DNA be removed, as was pointed out when the structure of DNA was determined [1] . In the Escherichia coli chromosome, ∼ 450,000 links need to be removed each generation, with the two type II topoisomerases, DNA gyrase and topoisomerase IV (TopoIV) being responsible for most of this unlinking. DNA gyrase acts preferentially to remove positive supercoiling that accumulates ahead of the replication fork, while TopoIV acts potentially both in front of and behind replication forks as they proceed [2] . Inactivation of TopoIV has little or no effect on growth or DNA replication rate, but prevents segregation of newly replicated sister loci and thus cell division, thereby demonstrating its essential role in decatenation [3] . An interaction between the ParC subunit of TopoIV and the structural maintenance of chromosomes (SMC) protein MukB has been inferred from live-cell imaging studies [4] and demonstrated in vitro [5] , [6] , [7] . Furthermore, this interaction can stimulate catalysis by TopoIV in vitro [5] , [6] , [8] and is predicted to promote decatenation in vivo [4] . MukBEF was first identified from a genetic screen designed to identify proteins that act in chromosome segregation [9] , and although it is unclear whether its primary role is in chromosome segregation or organization these functions are not mutually exclusive [10] . Functional fluorescent derivatives of MukBEF form foci that are normally associated with the replication origin region ( ori ) of the E. coli chromosome, and which have been proposed to position ori s before and after their replication, as well as recruiting TopoIV [4] , [11] , [12] . These foci contain on average eight dimers of dimer MukBEF complexes, hereafter termed MukBEF clusters, which adopt an ellipsoidal shape, with a mean diameter of ∼ 400 nm, irrespective of whether MukB, MukE or MukF was labelled [13] . Cluster association with ori requires that MukB can bind and hydrolyse ATP efficiently and that the ATPase heads can engage [13] . MukBEF complexes are restricted to some γ- and δ-proteobacteria, and have co-evolved with a subset of genes, including matP , whose product binds to multiple matS sites in the replication termination region ( ter) and organizes the Ter macrodomain [14] , [15] , [16] . Here we demonstrate an interaction between E. coli MukB and MatP by ChIP-seq, in vitro biochemistry and an in vivo two-hybrid analysis. Cells lacking MatP show a stable association of both ori and ter with positioned MukBEF clusters, consistent with MatP directing the displacement of wild-type MukBEF complexes from ter . This dispacement, which is impaired when MukB ATP hydrolysis is compromised, thereby facilitates MukBEF cluster association with ori . Cells lacking MatP show precocious ter segregation, which is delayed when the TopoIV-MukBEF interaction is impaired. We propose that the interplay between MukBEF and MatP directs the positioning of the chromosome with respect to MukBEF clusters and their associated TopoIV, thereby ensuring normal chromosome organization, and timely unlinking and segregation. ATPase-impaired MukB EQ EF complexes form clusters at ter Wild-type MukBEF complexes form clusters of molecules, revealed as fluorescent foci that associate with ori in steady-state cells when functional derivatives of MukB, MukE or MukF were fluorescently labelled and expressed from their endogenous promoters ( Fig. 1a ; refs 11 , 12 ). To assess this association quantitatively, we measured the shortest distance between a MukBEF centroid and the centroid of the fluorescent repressor-bound ori1 locus, located 15 kb CCW of oriC ( Fig. 1c ). This showed that in 86% of cells the distance between a MukBEF centroid and an ori1 focus centroid was ≤258 nm (2 pixels). This distance was used to define ‘colocalization’, a descriptive term that does not imply an interaction between MukBEF clusters and any specific sequence in the chromosome. 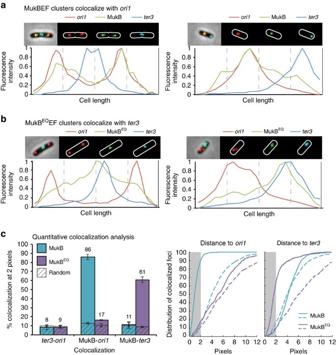Figure 1: ATP hydrolysis-impaired MukBEQEF complexes associate withter. Localization ofori1,ter3, and MukB-mYPet (SN182) (a) or MukBEQ-mYPet (SN311) (b). Theori1locus is alacOarray bound by LacI-mCherry, and theter3locus is atetOarray bound by TetR–CFP. The normalized fluorescence intensity along the cell length is shown below each image. (c) Left panel: % colocalization at 2 pixels between MukB, MukBEQ,ori1andter3focus centroids in the combinations shown. Dashed boxes represent the distances measured to a random pixel position in the cells analysed. The histograms show the mean (±s.d.) of three independent experiments. Middle and right panels show cumulative distributions of the distances between MukB, or MukBEQ, andori1orter3foci, respectively, obtained in one experiment. Dashed lines represent distances measured to a random pixel. The grey rectangle indicates the distances within 2 pixels (258 nm). See alsoSupplementary Figs 1 and 2. CFP, cyan fluorescent protein). Figure 1: ATP hydrolysis-impaired MukB EQ EF complexes associate with ter. Localization of ori1 , ter3 , and MukB-mYPet (SN182) ( a ) or MukB EQ -mYPet (SN311) ( b ). The ori1 locus is a lacO array bound by LacI-mCherry, and the ter3 locus is a tetO array bound by TetR–CFP. The normalized fluorescence intensity along the cell length is shown below each image. ( c ) Left panel: % colocalization at 2 pixels between MukB, MukB EQ , ori1 and ter3 focus centroids in the combinations shown. Dashed boxes represent the distances measured to a random pixel position in the cells analysed. The histograms show the mean (±s.d.) of three independent experiments. Middle and right panels show cumulative distributions of the distances between MukB, or MukB EQ , and ori1 or ter3 foci, respectively, obtained in one experiment. Dashed lines represent distances measured to a random pixel. The grey rectangle indicates the distances within 2 pixels (258 nm). See also Supplementary Figs 1 and 2 . CFP, cyan fluorescent protein). Full size image When we analysed a mukB[E1407Q ] mutant, whose protein product (hereafter, MukB EQ ) binds ATP, but is impaired in ATP hydrolysis [13] , [17] , [18] , [19] , we observed that the fluorescently labelled MukB EQ EF formed foci that colocalized with ter3 , a locus 50 kb CW of dif , irrespective of whether C-terminal green fluorescent protein, mYPet or mCherry fusions were used, and whether MukB EQ , MukE or MukF were labelled ( Fig. 1a–c ; ref. 13 ). Unlike wild-type MukBEF, we observed little or no ori1 colocalization with this mutant ( Fig. 1c ). Colocalization of MukB EQ EF and ter3 , occurred when ter3 was at midcell, where the divisome forms, or towards a cell pole, discounting the possibility that MukB EQ EF is divisome associated rather than directly with ter3 ( Fig. 1b ). Consistent with the ter3 association, MukB EQ EF focus-containing cells generally had a single focus, and quantitative analysis showed 61% colocalization between ter3 centroids and MukB EQ EF centroids ( Fig. 1b,c ; Supplementary Fig. 1 ). Cells expressing MukB EQ EF from the endogenous locus demonstrate all of the classical Muk − phenotypes—temperature-sensitive growth in rich medium, production of anucleate cells and a chromosome in which ori is mispositioned, as indicated by the decreased fraction of newborn cells with ori located at midcell and an increased fraction of cells with polar ori s when compared with the Muk + strain (compare Fig. 1a,b ; Supplementary Figs 1 and 2 ; refs 12 , 20 ). We showed that MukB EQ EF has residual ATPase activity that is ∼ 15% of that of the wild-type complex ( Supplementary Fig. 2d ), in agreement with that of Bacillus subtilis SMC complexes [17] , [21] . Consistent with this, molecules of MukB EQ EF in clusters had dramatically reduced turnover in a FRAP analysis, indicating that ATP hydrolysis is required for loading onto and/or dissociation from DNA [13] . Therefore, we explored the possibility that residual ATP hydrolysis by MukB EQ EF might be required for its association with ter , but insufficient for dissociation from ter and association with ori . To investigate this, we compared repletion of wild-type MukB and MukB EQ in cells that were otherwise MukB − E + F + . MukB or MukB EQ proteins were expressed from their normal chromosomal positions, but under the control of the P ara promoter rather than their endogenous promoter ( Fig. 2a ). The formation of MukBEF clusters was visualized after induction of expression, using MukE-mYPet ( Fig. 2 ; Supplementary Fig. 3 ). The increase in intensity of the brightest MukE pixel in cells was used to measure MukBEF focus formation, along with manual counting of MukBEF/MukB EQ EF focus number. Expression of wild-type MukB, led to a rapid and linear increase in pixel intensity for ∼ 20 min, mirrored by a concomitant increase in the fraction of cells with foci ( Fig. 2b ). The association of MukBEF foci with ori1 foci had approached the steady-state level after 20 min of repletion, when the relative positions of MukBEF and ori1 foci were almost identical to those in wild-type cells ( Supplementary Fig. 3 ). Longer repletion periods resulted in some aberrant focus positioning, indicative of excess MukB mirroring effects of MukBEF impairment, perhaps because excess MukB titrates out MukEF from functional complexes, consistent with other observations [22] . 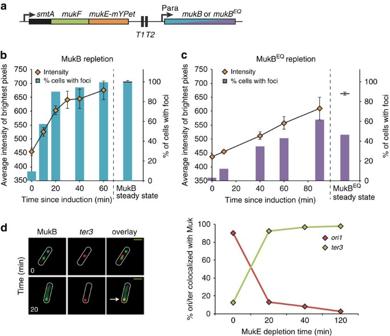Figure 2: MukBEQEF clusters form slowly. (a) Wild-type MukB or MukBEQwere expressed from an arabinose-inducible promoter at the chromosomalmukBlocus. Transcription from thesmtApromoter was blocked by terminators T1–T2. Repletion of wild-type MukB (AU2064) (b) and MukBEQ(AU2089) (c) in ΔmukBcells. Two methods were used to monitor focus formation; the average intensity of the brightest MukE-mYPet pixel in cells, as well as manual counting of foci (n=460–1,000 cells). Brightest pixel data are means (±s.e.m) of three experiments. Steady-state data were from cells where MukB/MukBEQwas expressed from their normal promoters. See alsoSupplementary Fig. 3. (d) MukBEF foci colocalize withterduring MukE depletion. MukBEF focus position was followed before (0) and after depletion. Left: snapshot images of cells with labelledter3and MukB are shown for the indicated depletion times. The arrow shows colocalization of MukB withteron MukE depletion. Right: %ori1(Ab86) orter3(Ab227) foci associated with a MukB focus, in cells with MukBEF foci, were plotted for each time point. After 80 min of depletion, cells had only weak MukBEF foci.n≥300. Figure 2: MukB EQ EF clusters form slowly. ( a ) Wild-type MukB or MukB EQ were expressed from an arabinose-inducible promoter at the chromosomal mukB locus. Transcription from the smtA promoter was blocked by terminators T1–T2. Repletion of wild-type MukB (AU2064) ( b ) and MukB EQ (AU2089) ( c ) in Δ mukB cells. Two methods were used to monitor focus formation; the average intensity of the brightest MukE-mYPet pixel in cells, as well as manual counting of foci ( n =460–1,000 cells). Brightest pixel data are means (±s.e.m) of three experiments. Steady-state data were from cells where MukB/MukB EQ was expressed from their normal promoters. See also Supplementary Fig. 3 . ( d ) MukBEF foci colocalize with ter during MukE depletion. MukBEF focus position was followed before (0) and after depletion. Left: snapshot images of cells with labelled ter3 and MukB are shown for the indicated depletion times. The arrow shows colocalization of MukB with ter on MukE depletion. Right: % ori1 (Ab86) or ter3 (Ab227) foci associated with a MukB focus, in cells with MukBEF foci, were plotted for each time point. After 80 min of depletion, cells had only weak MukBEF foci. n ≥300. Full size image The rate of formation of MukB EQ EF clusters was 3.8-fold (brightest pixel) to 6.2-fold (fraction of cells with foci) slower than for wild-type MukBEF clusters. This result indicates that the ∼ 15% residual ATP hydrolysis by MukB EQ EF is necessary for loading onto ter , and is consistent with the requirement of ATP hydrolysis for stable association of other SMC complexes with DNA [18] , [21] . We also showed that MukB-mYPet labelled clusters relocated from ori (95% colocalization at 0 min) to ter (98% colocalization at 20 min), as MukE was depleted by degron degradation ( Fig. 2d ), indicating that depletion of MukE has a regulatory consequence on MukBEF action, mirroring the MukB EQ EF ter association phenotype. We propose that cycles of ATP binding and hydrolysis by wild-type MukBEF are required for the steady-state association of its clusters with ori , consistent with the FRAP analysis [13] . In contrast, a low level of ATP hydrolysis by MukB EQ EF complexes is sufficient for a slow but stable association with ter , but not sufficient for the cycles of ATP-binding and hydrolysis required for the o ri association. The following sections reveal the molecular basis of these contrasting behaviours. MukBEF associates with MatP-bound matS sites The contrasting cellular localization patterns of wild-type MukBEF clusters with those of MukB EQ EF, and those of wild type during MukE depletion, led us to analyse the association of these complexes with the E. coli chromosome using ChIP-seq [23] , [24] , [25] , with FLAG-tagged MukB derivatives. Although wild-type MukBEF forms clusters associated with ori1 , we observed no significant enrichment at specific ori regions by ChIP-seq ( Supplementary Fig. 4 ). Highly transcribed genes gave similar signals for MukB, MukB EQ , MukB DA and MatP ( Supplementary Fig. 4 and Supplementary Fig. 5a ), most likely because single-stranded DNA present in these regions is highly reactive to formaldehyde [26] . Although enrichment at transfer RNA (tRNA) and ribosomal RNA genes has been shown for eukaryote and B. subtilis SMC proteins [18] , [27] , [28] , tRNA genes have been reported as false positives in yeast [29] . We have no basis for ascribing functional significance to the MukB signals in ori and note that unlike B. subtilis SMC, which interacts with ParB bound to parS sites, as well as to highly transcribed regions, ParB- parS is absent in E. coli , and we observed no signals that could be attributed to parS -like sequences. In contrast, when we analysed the enrichment pattern of MukB EQ , we observed specific signals in ter ( Fig. 3a ), consistent with the imaging analysis that shows that MukB EQ EF is ter associated ( Fig. 1 ). The peaks obtained within ter were centred at matS sites, as revealed by motif search and by comparison of the enrichment pattern of Flag-tagged MatP and MukB EQ ( Fig. 3a,b ; Supplementary Fig. 5b ; ref. 15 ). In addition, the absence of MukB EQ enrichment at ter in ΔmatP cells shows that the signals are MatP dependent, suggesting a physical interaction between the two proteins ( Fig. 3 ). 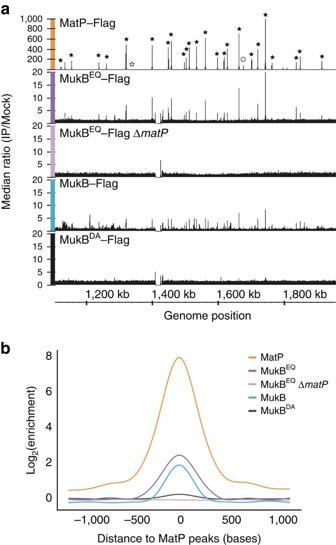Figure 3: MukBEQ–Flag protein enrichment atmatSsites is dependent on MatP. (a) Distribution of ChIP-seq signals interfor MatP–Flag, MukBEQ–Flag, MukBEQ–Flag ΔmatP, MukB–Flag and MukBDA–Flag. Each graph represents the ratio of the median number of reads of three experiments between Flag-tagged strains (IP) and untagged strains (Mock). Black stars indicate the positions ofmatSand pseudomatSsites and the circle indicates a non-mats-enriched region included in the analysis inb.matS5, which showed no enrichment, was not included into the analysis inb, and is indicated by a white star. The figure was generated using Integrated Genome Browser56. (b) Median signals of normalized samples (see experimental procedures), smoothed in a window of 2 kb centred to the position of the 26 most significant MatP peaks (indicated ina) are shown. The graph shows∼1.5-fold change between MukB and MukBEQ. Flat signals obtained for MukBEQ–Flag ΔmatPand MukBDA–Flag are indicative of an absence of significant enrichment. See alsoSupplementary Figs 4 and 5. Figure 3: MukB EQ –Flag protein enrichment at matS sites is dependent on MatP. ( a ) Distribution of ChIP-seq signals in ter for MatP–Flag, MukB EQ –Flag, MukB EQ –Flag Δ matP , MukB–Flag and MukB DA –Flag. Each graph represents the ratio of the median number of reads of three experiments between Flag-tagged strains (IP) and untagged strains (Mock). Black stars indicate the positions of matS and pseudo matS sites and the circle indicates a non- mats -enriched region included in the analysis in b . matS 5, which showed no enrichment, was not included into the analysis in b , and is indicated by a white star. The figure was generated using Integrated Genome Browser [56] . ( b ) Median signals of normalized samples (see experimental procedures), smoothed in a window of 2 kb centred to the position of the 26 most significant MatP peaks (indicated in a ) are shown. The graph shows ∼ 1.5-fold change between MukB and MukB EQ . Flat signals obtained for MukB EQ –Flag Δ matP and MukB DA –Flag are indicative of an absence of significant enrichment. See also Supplementary Figs 4 and 5 . Full size image By analysing the 26 chromosomal positions that gave the highest MatP enrichment, of which 21 were matS sites ( Fig. 3a , Supplementary Fig. 5c ), we observed that wild-type MukBEF exhibited a significant enrichment at these sites, while the ATP-binding deficient MukB DA mutant, which showed no evidence of an association with specific regions of the chromosome by live-cell imaging [13] , was not enriched ( Fig. 3b , Supplementary Fig. 5c ). This indicates that MukB and MukB EQ functionally interact with MatP- matS and are most likely loaded onto DNA in reactions that require ATP binding and hydrolysis. We propose that the relatively stable association of the ATP hydrolysis-impaired MukB EQ protein with MatP-bound matS sites reflects the fact that efficient release of MukBEF from ter requires ongoing cycles of ATP hydrolysis. Since duplex DNA is unreactive to formaldehyde in vitro [26] , the DNA distortion induced by MatP-binding to matS [30] will enhance the formaldehyde sensitivity of matS sites in MatP + cells. We therefore considered whether the MukBEF signals at matS arise because MatP-bound matS sites are formaldehyde reactive and that MukBEF is distributed over all of ter , without any specific association with MatP. We address these alternatives in the following section. MatP interacts with MukB in vivo and in vitro Since a candidate for MatP dimer binding to MukBEF was the dimeric MukB hinge, we tested for a MatP-hinge interaction in vivo by a bacterial two-hybrid assay [31] and in vitro using size exclusion chromatography and co-immunoprecipitation ( Fig. 4 ). In the two-hybrid analysis, the MukB dimerization hinge along with 172 amino acids of associated coiled-coil (hereafter called Hinge, Fig. 4a ) was tested for interactions with MatP and two truncation derivatives, of 18 and 20 C-terminal amino-acid residues (MatPΔC18 and MatPΔC20, respectively), that are unable to tetramerize [30] . We observed weak interaction signals between the Hinge and each of the MatP derivatives; these could reflect transient or weak interactions that do not require the MatP tetramerization domain ( Fig. 4b ). Strong signals were obtained between all combinations of MatP derivatives and between the Hinge derivatives, consistent with MatP and Hinge, each forming homodimers ( Supplementary Fig. 6a ). 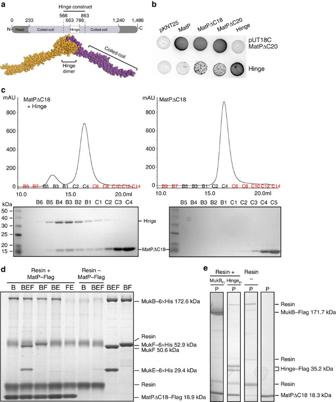Figure 4: MukB and MatP interactin vivoandin vitro. (a) Top: schematic of MukB protein. The Hinge construct carries residues 566–863. Bottom: space-filling representation of a dimer6containing most of the residues (572–854) of the Hinge construct. (b) The bacterial two-hybrid analysis is based on functional adenylate cyclase reconstitution31. Proteins of interest, as indicated, were fused to the N and the C terminus of the T25 and T18 domains, respectively. Blue colouring on X-gal plates reveals positive interactions. See alsoSupplementary MethodsandSupplementary Fig. 6afor all combinations in MatP+and ΔmatPcells. (c) Size exclusion chromatography of MatPΔC18 alone (right panel), or present at seven-fold molar excess over Hinge (left panel). The elution fractions indicated in black were analysed on SDS–PAGE; shown below each graph. Because of space constraints, not all fractions are shown in the upper panels. Also seeSupplementary Fig. 6b,c. (d) Co-Immunoprecipitation assay using resin-bound MatP–Flag, derived from over-expressed cell extracts, to assay for binding of MukB (Lane 1), MukBEF (Lane 2), MukBF (Lane 3), MukBE (Lane 4) and MukFE (Lane 5). MukB (Lane 6) and MukBEF (Lane 7) show no binding to the resin. Purified MukBEF (Lane 8) and MukBF (Lane 9), as used in the assay. The MW of the proteins used were: MukB-6 × His 172.6 kDa; MukF-6 × His 52.9 kDa; MukF 50.6 kDa; MukE-6 × His 29.4 kDa and MatPΔC18–Flag 16.9 kDa. (e) Co-immunoprecipitation shows MatPΔC18 is retained by MukB–Flag (lane 1) and Hinge–Flag (lane 2) attached to the anti-FLAG resin but not by the resin alone (lane 3). Lane 4: purified MatPΔC18-6 × His. Hinge proteins gave 2 bands on SDS–PAGE, maybe because of proteolytic cleavage. The MW of the proteins was: MukB–Flag 171.7 kDa; Hinge–Flag 35.2 kDa; MatPΔC18-6 × His 18.3 kDa. The lanes were derived from the same gel (shown inSupplementary Fig. 6d). MW, molecular weight. Figure 4: MukB and MatP interact in vivo and in vitro . ( a ) Top: schematic of MukB protein. The Hinge construct carries residues 566–863. Bottom: space-filling representation of a dimer [6] containing most of the residues (572–854) of the Hinge construct. ( b ) The bacterial two-hybrid analysis is based on functional adenylate cyclase reconstitution [31] . Proteins of interest, as indicated, were fused to the N and the C terminus of the T25 and T18 domains, respectively. Blue colouring on X-gal plates reveals positive interactions. See also Supplementary Methods and Supplementary Fig. 6a for all combinations in MatP + and Δ matP cells. ( c ) Size exclusion chromatography of MatPΔC18 alone (right panel), or present at seven-fold molar excess over Hinge (left panel). The elution fractions indicated in black were analysed on SDS–PAGE; shown below each graph. Because of space constraints, not all fractions are shown in the upper panels. Also see Supplementary Fig. 6b,c . ( d ) Co-Immunoprecipitation assay using resin-bound MatP–Flag, derived from over-expressed cell extracts, to assay for binding of MukB (Lane 1), MukBEF (Lane 2), MukBF (Lane 3), MukBE (Lane 4) and MukFE (Lane 5). MukB (Lane 6) and MukBEF (Lane 7) show no binding to the resin. Purified MukBEF (Lane 8) and MukBF (Lane 9), as used in the assay. The MW of the proteins used were: MukB-6 × His 172.6 kDa; MukF-6 × His 52.9 kDa; MukF 50.6 kDa; MukE-6 × His 29.4 kDa and MatPΔC18–Flag 16.9 kDa. ( e ) Co-immunoprecipitation shows MatPΔC18 is retained by MukB–Flag (lane 1) and Hinge–Flag (lane 2) attached to the anti-FLAG resin but not by the resin alone (lane 3). Lane 4: purified MatPΔC18-6 × His. Hinge proteins gave 2 bands on SDS–PAGE, maybe because of proteolytic cleavage. The MW of the proteins was: MukB–Flag 171.7 kDa; Hinge–Flag 35.2 kDa; MatPΔC18-6 × His 18.3 kDa. The lanes were derived from the same gel (shown in Supplementary Fig. 6d ). MW, molecular weight. Full size image We confirmed that the signal obtained in vivo reflects a direct interaction between MukB and MatP by co-immunoprecipitation and size exclusion assays. In the size exclusion assays, to maximize size differences between the proteins, we used the Hinge (36 kDa) and MatPΔC18 (18 kDa). MatPΔC18 eluted in the same fractions as the Hinge, when the Hinge was present in the sample ( Fig. 4c , Supplementary Fig. 6b,c ). Specific MukB–MatP interactions were also demonstrated when MatPΔC18–Flag proteins, bound to anti-Flag resin, specifically retained purified MukB, as well as MukE and MukF when they were complexed with MukB ( Fig. 4d ). The reciprocal experiment, in which resin-bound MukB–Flag or Hinge–Flag was used to assay for MatPΔC18 binding led to the same conclusion ( Fig. 4e ). We conclude that the signals of MukB enriched at matS sites observed in ChIP-seq reflect a physical in vivo interaction between the MukB hinge region and MatP. MatP promotes displacement of MukBEF from ter Given that fluorescent MukBEF foci are normally ori -associated and show no ter colocalization ( Fig. 1c ), we investigated if the interaction with MatP influences the cellular localization of MukBEF clusters. In Δ matP cells, wild-type MukBEF foci showed a high level of colocalization with ter3 , as well as with ori1 ( Fig. 5a ). To confirm that the observed MukB- ter colocalization was not a consequence of increased ter mobility observed in the absence of MatP [15] , we repeated the analysis in matP ΔC 20 cells, which have lost the interactions between matS -bound MatP dimers, because MatPΔC20 is unable to tetramerize [30] , and which showed the increased ter mobility of Δ matP cells [30] . We infer that ter is no longer anchored to the divisome at midcell in these cells, because a range of assays suggests that MatPΔC20 is unlikely to interact with ZapB [30] , [32] . 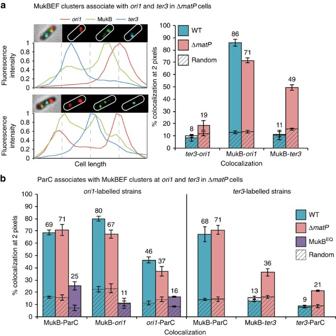Figure 5: Colocalization of MukBEF complexes with TopoIV andter. (a) Examples of colocalization of MukBEF withori1andter3in ΔmatPcells (left). ΔmatPcells have the same growth and cell cycle parameters as MatP+cells (Supplementary Methods). Histograms show the colocalization betweenori1,ter3and MukB-mYPet in ΔmatP(SN302, right).n>2,700 cells. Wild-type data fromFig. 1are shown for comparison. (b) Colocalization of MukB-mCherry, ParC-mYPet andori1in wild-type (ENOX5.130), ΔmatP(KK56) and MukBEQ(ENOX5.178) cells, orter3in wild-type (KK57) and ΔmatP(KK58) strains.n>2,400 cells. The brightest pixel was used to localize ParC-mYPet molecules within the cell4. The data represent the mean (±s.d.) of three independent experiments. The percentage represents colocalization in those cells that have foci. Note that ParC-mYPet MukBEQ-mCherry cells grew poorly. See alsoSupplementary Figs 7 and 8. Figure 5: Colocalization of MukBEF complexes with TopoIV and ter . ( a ) Examples of colocalization of MukBEF with ori1 and ter3 in Δ matP cells (left). Δ matP cells have the same growth and cell cycle parameters as MatP + cells ( Supplementary Methods ). Histograms show the colocalization between ori1 , ter3 and MukB-mYPet in Δ matP (SN302, right). n >2,700 cells. Wild-type data from Fig. 1 are shown for comparison. ( b ) Colocalization of MukB-mCherry, ParC-mYPet and ori1 in wild-type (ENOX5.130), Δ matP (KK56) and MukB EQ (ENOX5.178) cells, or ter3 in wild-type (KK57) and Δ matP (KK58) strains. n >2,400 cells. The brightest pixel was used to localize ParC-mYPet molecules within the cell [4] . The data represent the mean (±s.d.) of three independent experiments. The percentage represents colocalization in those cells that have foci. Note that ParC-mYPet MukB EQ -mCherry cells grew poorly. See also Supplementary Figs 7 and 8 . Full size image The pattern of colocalization of ori1 or ter3 with MukBEF in matP ΔC 20 cells was similar to that of MatP + cells ( Supplementary Fig. 7 ). Therefore, the observed ter3 association of MukBEF clusters in Δ matP cells is a direct consequence of MatP loss rather than an indirect effect arising from failure of tethering ter to the divisome, or from loss of MatP tetramerization-dependent condensation of ter . This association with ter in Δ matP cells suggests that the MukB–MatP interaction limits MukBEF cluster association with ter , either by limiting the accessibility to ter , or by promoting dissociation from ter . We favour the latter since MukB EQ EF associates with ter in MatP + cells, making it unlikely that accessibility to ter is an issue ( Fig. 1c ). MukB EQ EF clusters also remained associated with ter3 in Δ matP cells, albeit with a decrease in colocalization ( Supplementary Fig. 7 ). The difference in behaviour of MukBEF and MukB EQ EF with respect to their ter3 association in MatP + /Δ matP cells suggested that wild-type MatP bound to matS sites promotes release of MukBEF from ter . This displacement of MukBEF clusters by MatP must occur inefficiently or not at all with MukB EQ EF clusters at ter , because of reduced ATP hydrolysis by these complexes, and/or because of architectural differences between the MukBEF and MukB EQ EF complexes. We do not know the molecular mechanism that leads to the association between ter and MukBEF complexes in the absence of MatP. Nevertheless, the data clearly show that this MukBEF– ter association leads to an interaction of MukBEF with MatP bound to matS sites when MatP is present. We note also that MukBEF and MukB EQ EF clusters associated with ter in the absence of MatP, like MukBEF clusters at ori , gave no significant ChIP-seq signal, despite forming fluorescent foci in live-cell imaging. MukBEF–TopoIV interact independently of chromosome position As ParC associates with MukBEF clusters when they are positioned at ori ( Fig. 5b ; Supplementary Fig. 8 ; ref. 4 ), it was important to test whether this association was maintained when MukBEF clusters were at ter . The overall association between ParC and MukBEF clusters was the same in Δ matP and MatP + cells. Furthermore, ParC colocalized with both ter3 and ori1 in Δ matP cells, maintaining its association with MukBEF clusters at both positions ( Fig. 5b ). Therefore, the MukBEF–TopoIV interaction occurs independently of chromosomal position. In contrast, when we examined ParC colocalization with MukB EQ EF clusters at ter , we observed little ParC–MukB EQ EF association ( Fig. 5b ). This could be because DNA-bound MukB EQ EF molecules have a nucleotide state and/or architecture that fail to support stable ParC binding. Alternatively, stable association of MukB EQ EF with matS -site bound MatP could prevent ParC binding because MatP and ParC compete for binding to the MukB hinge. Irrespective of the mechanism, the nucleotide state of MukB EQ EF clusters loaded at ter influences directly, or indirectly, their association with TopoIV. MatP regulates MukBEF-stimulated TopoIV decatenation at ter Since our data showed that MukBEF accesses ter transiently in wild-type cells, and is more stably ter -associated in Δ matP cells, we tested if the presence of functional MatP and MukBEF influences TopoIV-mediated ter decatenation. In time-lapse experiments, we analysed the times between disappearance of DnaN foci at replication termination and ter3 segregation, and determined the time at which 50% of ter3 foci had segregated. Since ter3 replicates ∼ 2 min before most terminations at terC [3] and DnaN molecules take ∼ 5 min to unload at termination [33] , the measured time underestimates the time between ter3 replication and segregation by ∼ 7 min ( Fig. 6 and Supplementary Fig. 9a ). We therefore added 7 min to each of the measured values and defined this as ‘cohesion time’, which we propose reflects the time for newly replicated ter3 DNA to be decatenated. Consistent with this proposal, TopoIV availability at ori1 determines the time of ori1 segregation, with TopoIV overexpression reducing the segregation time of newly replicated ori1 loci from 14 to 5 min [3] . 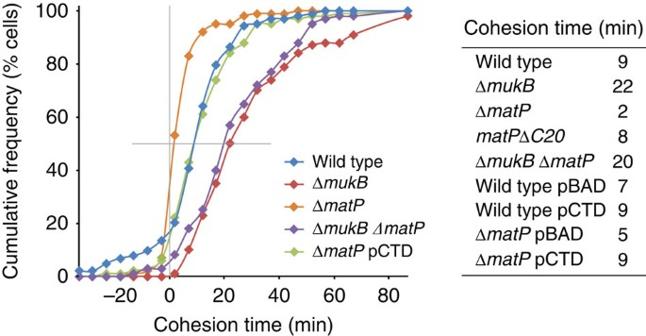Figure 6: MukBEF and MatP influencetersegregation. Time-lapse analysis of the time between replisome (DnaN-mCherry) disappearance andter3segregation.ter3replicates∼2 min before termination atterC, and DnaN takes∼5 min before it is unloaded after replication termination33; hence 7 min was added to the measured values to estimate ‘cohesion time’, which we define as the time for decatenation ofter3after its replication. Wild type, ENOX5.212; ΔmukB, AU2047; ΔmatP, AU2120; ΔmatPΔmukB, AU2125; ΔmatPpCTD, AU2157. n≥20. See also Methods andSupplementary Fig. 9. Figure 6: MukBEF and MatP influence ter segregation. Time-lapse analysis of the time between replisome (DnaN-mCherry) disappearance and ter3 segregation. ter3 replicates ∼ 2 min before termination at terC , and DnaN takes ∼ 5 min before it is unloaded after replication termination [33] ; hence 7 min was added to the measured values to estimate ‘cohesion time’, which we define as the time for decatenation of ter3 after its replication. Wild type, ENOX5.212; Δ mukB , AU2047; Δ matP , AU2120; Δ matP Δ mukB , AU2125; Δ matP pCTD, AU2157. n≥20. See also Methods and Supplementary Fig. 9 . Full size image Sister ter3 loci exhibited a 9-min cohesion time in wild-type cells, while Δ matP cells segregated precociously 2 min after ter3 replication ( Fig. 6 and Supplementary Fig. 9c ), consistent with an increase in the fraction of cells with 2 ter foci in Δ matP cells ( Supplementary Fig. 7a ), as reported previously [15] . An increased fraction of 2 ter cells could arise as either a consequence of an increased D period in the cell cycle, or because of a precocious early separation of sister loci after replication. Flow cytometry showed no evidence of an increased D period in Δ matP cells ( Supplementary Fig. 9d ; ref. 15 ), supporting the hypothesis of precocious segregation in Δ matP cells. Furthermore, because matPΔC20 cells have a wild-type ter segregation phenotype ( Fig. 6 and Supplementary Fig. 9c ), it seems unlikely that higher order tetramerization-dependent MatP- matS ‘condensed’ structures delay sister separation. Therefore we propose that the precocious separation of newly replicated ter loci observed in Δ matP cells is a direct consequence of the MukBEF–TopoIV interaction at ter stimulating decatenation, a related observation to the demonstration that increasing TopoIV enhances decatenation at ori1 (ref. 3 ). We then observed that Δ mukB cells had extended ter3 cohesion times of 20–22 min, irrespective of whether cells were MatP + or Δ matP , showing that the precocious separation in Δ matP cells is MukBEF dependent. As the ParC C-terminal domain (ParC-CTD) interacts with the MukB dimerization hinge [5] , [6] , [7] , we anticipated that ParC-CTD overexpression ( Supplementary Fig. 9b ) would impair the ParC–MukBEF interaction and thereby allow us to test if the requirement of functional MukBEF for timely ter segregation is a consequence of its role in recruiting and targeting TopoIV to ter . Overexpression of ParC-CTD in Δ matP cells led to a 4-min increase in cohesion time ( Fig. 6 ), consistent with MukBEF targeting TopoIV to preferred sites of action. In contrast, ParC-CTD overexpression did not reduce cohesion time in MatP + cells ( Fig. 6 and Supplementary Fig. 9c ). The data support the hypothesis that MatP displaces wild-type MukBEF clusters and their bound TopoIV molecules from ter , and that the MukBEF–TopoIV association with ter in Δ matP cells promotes decatenation. A corollary is that MatP, by displacing MukBEF and its associated TopoIV, prevents premature ter decatenation and segregation in MatP + cells. The difference in cohesion times obtained with ParC-CTD overexpression and deletion of the mukB gene could be a consequence of MukBEF having additional roles in ter segregation independently of TopoIV; for example, through chromosome positioning and/or organization. Alternatively, ParC-CTD may not compete effectively in preventing the MukBEF–ParC interaction, perhaps because this protein, unlike full-length ParC, is monomeric [34] . By using an interdisciplinary approach, we have revealed how MatP regulates the position and action of E. coli TopoIV and MukBEF, complexes that play sequential roles in chromosome unlinking and segregation. The work has demonstrated that MatP regulates the distribution of MukBEF and TopoIV on the nucleoid by displacing MukBEF clusters and their associated TopoIV from ter . During replication of the E. coli chromosome, precatenation links between sisters arise as replication proceeds when replisomes rotate [3] , [35] . Most of these are removed by the type II topoisomerase TopoIV, although the type I topoisomerase III can potentially decatenate regions of the chromosome that are single stranded; for example, immediately behind replication forks [36] . Furthermore, FtsK DNA translocase-dependent XerCD site-specific recombination at dif sites also leads to decatenation [37] . Catenation links are likely to form universally as replication proceeds, since catenane accumulation has been reported when type II topoisomerase activity is compromised in a number of systems [38] , [39] . MukBEF and other bacterial SMC complexes form clusters associated with ori [11] , [12] , [28] , [40] and have been proposed to promote segregation by positioning the newly replicated sister ori s [4] , or by ori condensation [41] . The demonstration that MukB interacts with the ParC subunit of TopoIV to promote catalysis in vitro [5] , [6] , [7] , and that fluorescent ParC forms foci associated with MukBEF clusters at ori in vivo [4] , suggested a functional link between the action of TopoIV in decatenation and the facilitation of chromosome segregation by MukBEF. We have now validated such a link by showing that MukBEF-directed association of TopoIV at ter influences its segregation efficiency, consistent with TopoIV availability influencing sister segregation timing [3] . We propose that this is a consequence of enhanced decatenation by TopoIV, because the MukBEF–TopoIV interaction stimulates catalysis [4] and/or leads to a higher local concentration of TopoIV in regions of the chromosome associated with MukBEF clusters. Similarly, a functional interaction between condensin and TopoII, the eukaryote orthologue of TopoIV, has been reported to aid decatenation in yeast [42] , while more generally, TopoII–condensin interactions have been proposed to be important for mitotic chromosome organization [38] , [43] , suggestive of evolutionary conserved associations and functions. The formation of ori -associated MukBEF clusters requires that MukBEF is able to bind and hydrolyse ATP [11] , [13] . The clusters contain on average eight heads-engaged MukB dimers of dimers, with a relative stoichiometry of MukB/E/F of 4:4:2 (ref. 13 ). MukB EQ EF also forms heads-engaged clusters in vivo with identical stoichiometry. In contrast, complexes with unengaged heads have the 2:4:2 stoichiometry predicted from biochemical studies [19] . Mutants that are unable to engage heads, or to bind ATP, do not form clusters as judged by the lack of fluorescent foci [13] ; similarly, the ATP-binding defective MukB DA , failed to give a MatP-dependent ChIP-seq signal at matS sites, reinforcing the view that loading of MukBEF complexes onto DNA requires ATP binding and hydrolysis. The slow rate of MukB EQ EF cluster formation at ter that we measured correlates with its residual ATPase activity and is consistent with a mechanism in which a low level of ATP hydrolysis is required for cluster formation at ter , but is insufficient for significant ori localization. The observation that MukBEF clusters associate with ter as MukE is depleted, mimicking the mukB EQ EF phenotype, is consistent with a regulatory role of MukE in MukBEF function [44] . We propose that MukB EQ EF clusters at ter have one or two molecules of ADP bound per MukB dimer, depending on whether one or two ATPs were hydrolysed during loading; in either case the observed stoichiometry would only result if the heads remained engaged as a consequence of failing to release product ADP and/or phosphate. We favour the hypothesis that one ATP is hydrolysed on loading, while the second is hydrolysed during unloading. This is consistent with the data here, and from our earlier work that showed that MukB EQ EF complexes are not readily dissociated from ter [13] . Understanding of the molecular changes that occur during cycles of ATP binding and hydrolysis is central to a molecular understanding of SMC action. The functional significance of the ter association observed when ATPase activity was compromised in mukB EQ cells, or when MukE was depleted, was reinforced when we demonstrated that in Δ matP cells both ori and ter colocalize with wild-type MukBEF clusters. The inferred in vivo interaction between MukB and MatP from the ChIP-seq analysis, and the subsequent demonstration of a direct interaction between the MukB hinge region and MatP led us to show that MatP modulates MukBEF complex activity and positioning ( Fig. 7 ). Therefore, MatP is not a loading factor for directing the association of MukBEF clusters with ter , in contrast to the cohesin loading factors Scc2-4 (ref. 45 ), and ParB bound to parS sites in B. subtilis [28] , [40] . The mechanisms that direct the association of MukBEF clusters with ori and ter remain obscure. The MukB EQ EF ChIP-seq signals at matS correlate well with the cytological association of clusters with ter . We assume that the failure to see wild-type MukBEF clusters at ter in MatP + cells by imaging is a consequence of the interaction of individual complexes being transient, yet sufficient to give a ChIP-seq signal. Our failure to identify specific binding of MukBEF to ori sequences is likely because the association does not distort the DNA sufficiently to make it formaldehyde sensitive and/or because MukBEF is associated with multiple unrelated DNA sequences in this region. Similarly the association of MukB EQ EF with ter in Δ matP cells gave no significant ChIP-seq signal in ter , presumably for the same reason. 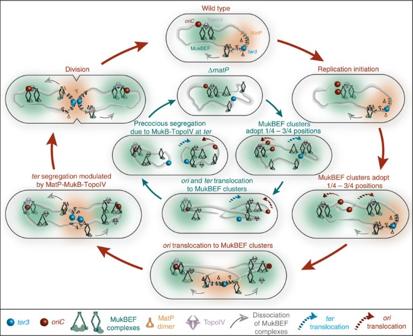Figure 7: Model of the interplay between MukBEF, TopoIV and MatP in chromosome positioning, unlinking and segregation. Outer circle (red arrows; clockwise from top). In wild-type newborn cells, MukBEF clusters and associated TopoIV are positioned at midcell by an unknown mechanism.oriassociates with these clusters. MukBEF complexes load onto DNA in ATP hydrolysis-dependent reactions. Complexes that encounter MatP-matSundergo ATP-hydrolysis-dependent dissociation fromter, thereby depleting theterregion from MukBEF whether in single complexes or in clusters, (and thereby facilitating theoriassociation). After replication initiation, MukBEF clusters localize to the nucleoid quarter positions, followed by the newly segregatedoris4. The process that directs theorito the MukBEF clusters is unknown, but appears to require multiple cycles of ATP binding and hydrolysis, could involve repeated interactions with the chromosome by a ‘rock-walker’13or ‘zipping’47,48mechanism, and may facilitate chromosome ‘organization’. Directional ‘zipping’ of the chromosome through MukBEF clusters, would result in active segregation or translocation of newly replicatedoristo the cell quarter positions. MukBEF complexes interact with TopoIV when not associated with MatP-matS, thereby enhancing decatenation other than in regions bound by MatP-matS. Inner circle (dark arrows; clockwise from top). In ΔmatPcells, the positioned MukBEF clusters associate withoriandter, because the lack of MatP prevents displacement ofterfrom MukBEF complexes. Consequently, the MukBEF–TopoIV interaction leads to enhanced decatenation atterand precocious segregation of newly replicatedters. Figure 7: Model of the interplay between MukBEF, TopoIV and MatP in chromosome positioning, unlinking and segregation. Outer circle (red arrows; clockwise from top). In wild-type newborn cells, MukBEF clusters and associated TopoIV are positioned at midcell by an unknown mechanism. ori associates with these clusters. MukBEF complexes load onto DNA in ATP hydrolysis-dependent reactions. Complexes that encounter MatP- matS undergo ATP-hydrolysis-dependent dissociation from ter , thereby depleting the ter region from MukBEF whether in single complexes or in clusters, (and thereby facilitating the ori association). After replication initiation, MukBEF clusters localize to the nucleoid quarter positions, followed by the newly segregated ori s [4] . The process that directs the ori to the MukBEF clusters is unknown, but appears to require multiple cycles of ATP binding and hydrolysis, could involve repeated interactions with the chromosome by a ‘rock-walker’ [13] or ‘zipping’ [47] , [48] mechanism, and may facilitate chromosome ‘organization’. Directional ‘zipping’ of the chromosome through MukBEF clusters, would result in active segregation or translocation of newly replicated oris to the cell quarter positions. MukBEF complexes interact with TopoIV when not associated with MatP- matS , thereby enhancing decatenation other than in regions bound by MatP- matS . Inner circle (dark arrows; clockwise from top). In Δ matP cells, the positioned MukBEF clusters associate with ori and ter , because the lack of MatP prevents displacement of ter from MukBEF complexes. Consequently, the MukBEF–TopoIV interaction leads to enhanced decatenation at ter and precocious segregation of newly replicated ters . Full size image We have shown that in the absence of MatP, wild-type MukBEF clusters at ter colocalize with ParC and this correlates directly with more efficient TopoIV-mediated ter decatenation in Δ matP cells ( Fig. 7b ). Modulation of TopoIV recruitment to ter by MukBEF and MatP may ensure sufficient cohesion time between newly replicated ter sisters, thereby helping coordinate the late stages of chromosome segregation with cell division. The observation that Δ mukB cells are more delayed in ter segregation than when the MukB-ParC interaction is impaired, indicates that MukBEF may have additional roles in ter segregation, such as positioning and/or organization, as proposed for ori [4] . The results here, taken together with previous results of ourselves, and others, lead to the model depicted in Fig. 7 . MukBEF complexes form positioned clusters on the nucleoid. The molecular basis for forming a cluster from MukBEF complexes is unknown, as is the positioning mechanism, but this superficially resembles the ParAB- parS systems that position replication origins and large protein machineries at fixed positions on the nucleoid (most commonly at mid-nucleoid and quarter positions) [46] . In steady-state cells these clusters act to exclusively position the replication origin region of the chromosome, a process dependent on the role of MatP- matS in displacing ter from MukBEF clusters. We propose that MukBEF complexes are loaded onto different parts of the chromosome, with preferential loading within ter , based on the ter localization of clusters of MukB EQ EF, and of MukBEF when MatP is absent or MukE depleted. MukB EQ EF clusters, which associate slowly with ter , apparently as a consequence of their impaired ATP hydrolysis, are dissociated poorly by MatP from ter , indicating a requirement of ATP hydrolysis for release from ter and subsequent association between ori and these clusters. This apparent requirement of ATP hydrolysis for ter association and dissociation, which is consistent with FRAP data [13] , supports the hypothesis that only one of the two ATPs bound to a MukB dimer are hydrolysed in each step. The MatP-stimulated dissociation between wild-type MukBEF complexes and ter is apparently a requisite for subsequent exclusive association of clusters with ori . We propose that MukBEF complexes, whether in clusters or not, frequently transiently associate with ter . MatP- matS -promoted displacement from ter leads to clusters becoming excluded from ter , thereby facilitating ori association. We propose that multiple cycles of ATP binding and hydrolysis lead to translocation of MukBEF complexes in clusters with respect to the chromosome, analogous to the way that SMC complexes in B. subtilis have been proposed to ‘zip along the chromosome’ after loading at ori through interaction with ParB- parS [47] , [48] . Such a translocation could act to actively direct ori to postioned MukBEF clusters. During this proposed transit, they may act as ‘condensins’, since MukBEF is implicated in global chromosome organization as well as in ori positioning. By associating with TopoIV, the MukBEF complexes may direct decatenation activity to those regions of the nucleoid with which MukBEF interacts transiently or more stably. The work here has highlighted the complexity of the interaction network necessary for the cell to ensure the coordination of processes responsible for chromosome organization and segregation. The organization, replication and segregation choreography of the E. coli chromosome in which the newly replicated origins move from the centre of the cell to the quarter positions, and ter migrates from the new pole to midcell to replicate [46] , [49] , implies an active positioning of ori and ter , mediated by MukBEF and MatP, respectively. The interaction between MukB and MatP, demonstrated here, brings new insight by linking ori and ter , opposite regions of the chromosome, which reside at different cellular positions for most of the cell cycle. This interplay is likely to play a central role in coordinating the early and late stages of segregation by determining the relative positions of MukBEF clusters with respect to ori and ter , thereby helping deliver TopoIV differentially to ori and ter , influencing decatenation activities spatially. Bacterial species that have MukBEF rather than typical SMC complexes also have MatP, indicative of their co-evolved functional dependence, and reinforcing their collaboration highlighted here. As insight into the organization of bacterial chromosomes is becoming more complete, it seems there are a number of variations on common themes [50] . Future work is needed to understand the implications of having a ter-ori -coordinated organization in E. coli (with MukBEF–MatP- matS as key players), rather than the ori -coordinated (using SMC-ParAB- parS ) organization found in bacteria in which newborn cells have ori at one pole and ter at the other. Bacterial strains and plasmids and growth Strains and plasmids used in this study are listed in Supplementary Table 1 and 2 , respectively. A description of the constructions is in Supplementary Methods . Unless otherwise stated, cells were grown at 30 °C in M9 glycerol (0.2%) supplemented with required amino acids (threonine, leucine, proline, histidine and arginine—0.1 mg ml −1 ) to an A 600 of 0.05–0.2 before imaging. Generation times for all strains were ∼ 170 min under these conditions. Construction of the MukB repletion strains The MukB repletion system is similar to that used for MukF repletion [11] , however, rather than inducing MukB expression from an ectopic locus the inducible mukB gene was introduced at its natural chromosomal locus. The P ara promoter from pBAD24 was introduced upstream of mukB with the T1–T2 transcriptional terminators [51] from the rrnB operon upstream of this to limit transcriptional readthrough from the smtA promoter ( Fig. 2a ). When grown in glucose there should be no induction of mukB gene expression and the cells should have a Muk − phenotype. The wild-type araC gene has also been re-introduced into the repletion strains to allow control of the P ara promoter. The strains carry ΔaraBAD so that arabinose will not be metabolized. Live-cell imaging Cell cultures were spotted onto an M9-gly 1% agarose pad on a slide. Images were taken using a × 100 oil immersion objective (Nikon Plan Apo × 100 1.40 PH3 DM) on a Nikon Eclipse TE2000-U microscope, equipped with a CoolSNAP HQ [2] CCD camera (Photometrics). MetaMorph software was used for image acquisition. Image analysis For the semiquantitative analysis of fluorescence distributions, fluorescence distributions in cells were plotted as line profiles using the Plot profile command of Fiji. Fluorescence intensity was normalized between 0 and 1. For the quantitative analysis of focus localization and colocalization, detection of MukB, ori1 and ter3 foci was done manually using MicrobeTracker tool SpotFinderM [52] . Custom MATLAB scripts were used to extract the numbers and position of foci [53] , and to measure the shortest distance per cell between two spots (the method described in ref. 4 was modified for manually identified spots), and are available on request. In ParC-labelled strains, the analysis used the method described in ref. 4 . MukB, ori1 and ter3 foci were detected automatically by Gaussian fitting, and the brightest pixel was used as to define a ParC focus. Data were then adjusted to represent only the fraction of cells with foci. For the analysis of focus formation during repletion, we employed two independent methods for monitoring MukBEF focus formation using MukE-mYPet. First of all, we manually counted MukBEF foci. Second, after using MicrobeTracker to identify cells, we used a bespoke Matlab script [4] to identify and record the intensity of the brightest mYPet pixel in every cell. The brightest pixel represents the point in the cells where fluorescent MukE-mYPet molecules have the highest residence time and thus where foci are forming. It should be noted that while MukBEF can form multiple foci within cells, the brightest pixel finds exactly one pixel with the highest intensity for MukBEF. The brightest pixel data represented in Fig. 2b,c has been adjusted to take into account that while 99% of wild-type cells have a MukBEF focus, only 47% of mukB EQ cells have a MukB EQ EF focus in steady-state growth. MukB repletion in steady-state cells Cells were grown overnight in M9 glucose at 30 °C to an A 600 of 0.05. A 1 ml sample was taken, additional glucose was added to 0.2% to ensure repression of P ara - mukB and incubation continued at 30 °C for 2 h. A sample of cells (0 min) was taken and imaged before beginning the repletion. For repletion, the cells were spun down and resuspended in M9 glycerol plus 0.2% arabinose. Samples were taken at 0, 10, 20, 30, 40 and 60 min after induction of repletion and in the case of the MukB EQ repletion an additional sample was taken at 90 min. All samples were spotted onto a pre-warmed M9-gly 1% agarose pad on a slide and imaged using the microscope. Terminus segregation in steady-state cells Cells were grown overnight in M9 glycerol at 30 °C to an A 600 of 0.05. A 1 ml sample was taken and IPTG was added to a concentration of 0.5 mM and incubated for 60 min at 30 °C. IPTG was added to induce expression of TetR-mCerulean to visualize the ter3 array. Samples were spotted onto a pre-warmed M9-gly, 0.5 mM IPTG, 1% agarose pad on a slide and imaged in time-lapse at 30 °C. Cells were imaged every 5 min for 2 h. For analysis of asynchronously growing cells, the timing of disappearance of the replisome (mCherry-DnaN) and of ter3 segregation was recorded. We observed that ter3 foci can transiently separate and associate immediately after replication, presumably as a consequence of precatenation links allowing transient sister separation; hence we defined complete ter3 separation as the point on which the foci remained separate for three consecutive 5-min time points. The robustness of the assay is indicated by the small variance in ‘cohesion times’ ( Fig. 6 ; Supplementary Fig. 9a ) for a given strain as indicated by the rapid increases in 2- ter3 focus cells. The assay interpretations assume that the different cohesion times arise from changes in segregation (decatenation) time rather than changes in time of DnaN focus disappearance. Bacterial two-hybrid assay The bacterial two-hybrid assay is based on functional adenylate cyclase T18 and T25 domain reconstitution [54] . Consequent cAMP synthesis allows transcription of the lactose operon, visualized as a blue colour on X-gal indicator plates. Cells were co-transformed with pKNT25 and pUT18C plasmids expressing the proteins indicated fused to the N terminus of the T25 domain and the C terminus of the T18 domain, respectively. Co-transformation with empty plasmids was used for negative controls. Cells were incubated at 30 °C for 2 days on an LB plate containing 100 μg ml −1 ampicillin and 50 μg ml −1 kanamycin. For each transformation, 5–6 clones were resuspended in LB containing 50 μg ml −1 ampicillin, 50 μg ml −1 kanamycin and 0.5 mM IPTG and spotted on LB plates containing 50 μg ml −1 ampicillin, 50 μg ml −1 kanamycin, 0.5 mM IPTG and 60 μg ml −1 or 120 μg ml −1 X-gal. After an overnight incubation at 30 °C, plates were incubated in the dark at room temperature for 2 to 4 days to allow the colour to develop. Each transformation was performed at least three times, leading to the same overall conclusions. ChIP-seq Cells were grown in LB at 37, or 22 °C for mukB mutant derivatives, to an A 600 of 0.5, and cross-linked with 1% formaldehyde for 20 min at 22 °C. The reaction was then quenched with 500 mM glycine. The equivalent of 250 ml of cells at an A 600 of 0.5 was harvested by centrifugation at 5,200 g for 30 min, washed twice with Tris-buffered-saline (pH 7.5), resuspended in 1 ml of lysis buffer (10 mM Tris (pH 7.5), 20% sucrose, 50 mM NaCl, 10 mM EDTA, 10 mg ml −1 of lysozyme, 0.1 mg ml −1 RnaseA) and incubated at 37 °C for 30 min. Following lysis, 4 ml of immunoprecipitation buffer (50 mM HEPES-KOH (pH 7.5), 150 mM NaCl, 1 mM EDTA, 1% Triton X-100, 0.1% sodium deoxycholate, 0.1% SDS) and phenylmethylsulfonyl fluoride (final concentration of 1 mM) was added. Cellular DNA was sheared by sonication to an average size of 200–1,000 bp. Cell debris was removed by two centrifugation steps at 16,620 g for 5 min. About 900 μl of the supernatant was used for each immunoprecipitation experiment. The sample was incubated with 2 μl of anti-Flag M2 Monoclonal Antibody (Sigma F3165) for 1 h at room temperature on a rotating wheel. Then 80 μl of DynabeadsProteinG (Life Technology) were added and incubated for 15 h at 4 °C. The beads were separated from samples by using DynaMag-2 magnet (Life Technology), and washed twice with immunoprecipitation buffer (as above), once with immunoprecipitation buffer containing 500 mM NaCl, once with wash buffer (10 mM Tris-HCl (pH 7.5), 250 mM LiCl, 1 mM EDTA, 0.5% IGEPAL CA-630, 0.5% sodium deoxycholate) and once with Tris-EDTA buffer (pH 7.5). Immunoprecipitated complexes were then removed from the beads by treatment with 100 μl of elution buffer (50 mM Tris-HCl (pH 7.5), 10 mM EDTA, 1% SDS) at 65 °C, with shaking at 1,400 r.p.m. for 30 min. Uncross-linking was achieved by addition of 90 ng μl −1 of proteinase K and incubation for 15 h at 50 °C followed by 4 h at 65 °C. DNA was purified using Purelink PCR Micro Kit (Invitrogen). Sequencing was performed on an Illumina HiSeq 2000 platform (Oxford Genomics Centre, Wellcome Trust Center For Human Genetics). Reads were mapped to the MG1655 reference genome and the data deposited at NCBI Omnibus [55] . See Supplementary Methods for details of the analysis. Biochemical assays Recombinant proteins were subcloned into a pET vector, expressed and purified from E. coli C3013I. Details can be found in the Supplementary Methods . For co-immunoprecipitation assays, fresh cell lysates carrying FLAG-tagged MatPΔC18, MukB or Hinge were prepared in buffer containing 50 mM HEPES pH 7.5, 300 mM NaCl, 5% glycerol supplemented with a protease inhibitor tablet. About 10 ml of lysates were mixed with 150 μl anti-Flag M2 Affinity gel (Sigma-Aldrich), incubated for 1 h at 4 °C. The resin was then washed three times with same buffer containing 250 mM NaCl, resuspended in 1 ml of buffer I (50 mM HEPES pH 7.5, 100 mM NaCl), and purified MukB, MukE, MukF or MatPΔC18 was added as indicated. After 45-min incubation (4 °C) the resin was washed three times, resuspended in 200 μl of protein loading buffer (NEB) and analysed on 4–20% gradient SDS–PAGE. For size exclusion chromatography, purified proteins were fractionated on a Superose 6 10/300 GL column equilibrated with 50 mM HEPES, pH 7.5 buffer containing 100 mM NaCl, 1 mMDTT, 1 mM EDTA, 5 mM MgCl 2 at a flow rate of 0.5 ml min −1 . About 500 μl samples containing MatPΔC18 (73 μM) and/or Hinge (15 μM), were injected on the column and run at flow rate of 0.5 ml min −1 . About 500 μl fractions were collected and analysed on 4–20% gradient SDS–PAGE. Accession codes: ChiP-seq data are available in the NCBI’s Gene Expression Omnibus 55 , series accession number GSE67221 . How to cite this article: Nolivos, S. et al . MatP regulates the coordinated action of topoisomerase IV and MukBEF in chromosome segregation. Nat. Commun . 7:10466 doi: 10.1038/ncomms10466 (2016).